Self-shaping composites with programmable bioinspired microstructures Shape change is a prevalent function apparent in a diverse set of natural structures, including seed dispersal units, climbing plants and carnivorous plants. Many of these natural materials change shape by using cellulose microfibrils at specific orientations to anisotropically restrict the swelling/shrinkage of their organic matrices upon external stimuli. This is in contrast to the material-specific mechanisms found in synthetic shape-memory systems. Here we propose a robust and universal method to replicate this unusual shape-changing mechanism of natural systems in artificial bioinspired composites. The technique is based upon the remote control of the orientation of reinforcing inorganic particles within the composite using a weak external magnetic field. Combining this reinforcement orientational control with swellable/shrinkable polymer matrices enables the creation of composites whose shape change can be programmed into the material’s microstructure rather than externally imposed. Such bioinspired approach can generate composites with unusual reversibility, twisting effects and site-specific programmable shape changes. Incorporating programmable shape change into synthetic materials enables enticing technologies that respond to environmental changes ranging from sun-following solar panels to reactive textiles to morphing building features. A variety of synthetic materials have been developed for applications requiring shape changes, including, for example, NiTi metallic alloys, photomechanical polymeric and composite films [1] , [2] , [3] , and thermoplastic polyurethanes [4] . However, the basic mechanism leading to shape changes in these materials are very specific to their chemical composition, which limits the functionalities achievable. For example, the shape-memory effect in NiTi alloys is caused by a reversible martensitic transformation of the metal’s crystalline structure. Likewise, photomechanical systems require specific light-sensitive liquid crystalline polymers [1] , [2] , [3] , and polyurethanes rely on the combination of hard and soft polymeric domains to change shape under external stimulus. Other shape-changing synthetic systems have been created, including, for example, sheets with origami-like folding properties produced either by lithographically depositing multiple layers of different materials [5] , [6] , [7] or by introducing electrically accessible actuators in specific regions of the sheet [8] . While the resulting heterogeneous structures lead to unique autonomous folding effects, the isotropic nature of the materials involved and the uniform thickness of the layers produced limit the shape changes to bending movements. Moreover, the preparation of self-folding films through lithographic processes involves numerous deposition steps and leads to stress-concentrating sharp interfaces that are susceptible to delamination. Shape-changing materials are not very prevalent in synthetic systems but are widespread in nature, particularly in plants [9] , [10] , [11] , [12] , [13] , [14] , [15] , [16] , [17] , [18] . Because of the limited chemical resources and processing conditions, plants have evolved mechanisms that rely on their internal heterogeneous architecture to achieve shape change upon external stimulus [9] , [10] , [11] , [12] . Hydration-triggered shape change in natural systems offers a passive, yet dramatic, response with only changes in surrounding humidity levels and is exhibited in diverse seed dispersal units, such as pinecones, wheat awn structures and orchid tree seedpods ( Supplementary Movie 1 ). In these three specific structures, various shape changes from bending to twisting are enabled depending on the architecture of stiff cellulose microfibrils (CMFs) within the extracellular matrices of the seed dispersal units ( Fig. 1 ). The basic concept underlying such shape-changing strategy is the restriction of swelling or shrinkage of the surrounding matrix in the direction of the reinforcing fibril [19] , [20] . The orientation of CMFs is defined by the angle between the fibres and the long axis of the cell, also known as the CMF angle. Recreating artificially the self-shaping strategy of natural materials could provide a more straightforward pathway towards three-dimensional (3D) manufactured materials with a wider variety of structurally programmable shape changes. 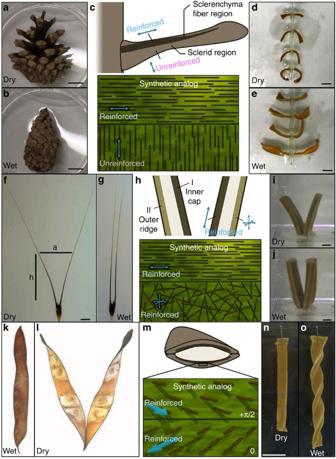Figure 1: Shape changes in natural seed dispersal units and synthetic reinforced composites before and after swelling. (a,b) A conifer pinecone (a) dried out and (b) fully hydrated. (c) Cartoon schematic indicating the predominant orientation of CMFs within a pinecone scale according to refs16,17. (d,e) Synthetic pinecone scales constructed by orienting UHMR platelets in a similar bilayer structure within gelatin shown (d) as-prepared and (e) fully hydrated. (f,g) A wheat awn system (f) dried out and (g) fully hydrated. Reprinted from ref.9(reproduced with permission from AAAS). (h) Cartoon schematic indicating the predominant orientation of CMFs within a wheat awn according to ref.9. (i,j) Synthetic wheat awn systems constructed by orienting magnetized alumina platelets in a similar bilayer structure within gelatin shown (i) as-prepared and (j) fully hydrated. (k,l) An orchid tree seedpod (k) hydrated and (l) dried out. Reprinted from ref.18(reproduced with permission from AAAS). (m) Cartoon schematic indicating the predominant orientation of CMFs within the orchid tree seedpod according to ref.18. (n,o) Synthetic chiral seedpods constructed by orienting UHMR platelets in a similar bilayer structure within gelatin shown (n) as-prepared and (o) fully hydrated. All scale bars are 1 cm. Figure 1: Shape changes in natural seed dispersal units and synthetic reinforced composites before and after swelling. ( a , b ) A conifer pinecone ( a ) dried out and ( b ) fully hydrated. ( c ) Cartoon schematic indicating the predominant orientation of CMFs within a pinecone scale according to refs 16 , 17 . ( d , e ) Synthetic pinecone scales constructed by orienting UHMR platelets in a similar bilayer structure within gelatin shown ( d ) as-prepared and ( e ) fully hydrated. ( f , g ) A wheat awn system ( f ) dried out and ( g ) fully hydrated. Reprinted from ref. 9 (reproduced with permission from AAAS). ( h ) Cartoon schematic indicating the predominant orientation of CMFs within a wheat awn according to ref. 9 . ( i , j ) Synthetic wheat awn systems constructed by orienting magnetized alumina platelets in a similar bilayer structure within gelatin shown ( i ) as-prepared and ( j ) fully hydrated. ( k , l ) An orchid tree seedpod ( k ) hydrated and ( l ) dried out. Reprinted from ref. 18 (reproduced with permission from AAAS). ( m ) Cartoon schematic indicating the predominant orientation of CMFs within the orchid tree seedpod according to ref. 18 . ( n , o ) Synthetic chiral seedpods constructed by orienting UHMR platelets in a similar bilayer structure within gelatin shown ( n ) as-prepared and ( o ) fully hydrated. All scale bars are 1 cm. Full size image We present a synthetic framework for building autonomous self-shaping composites in which the shape change is programmed within the microstructure of 3D macroscopic objects by controlling the local orientation of stiff reinforcing elements in a swellable/shrinkable surrounding matrix. To gain control over reinforcement architectures, we exploit the ultra-high magnetic response (UHMR) exhibited by discontinuous, anisotropic reinforcement microparticles coated with superparamagnetic iron oxide nanoparticles [21] . By applying weak external magnetic fields only during sample preparation, reinforcement particles can be oriented into architectures akin to the natural systems or into a wide range of completely unique and programmable shape-changing microstructures. To illustrate how the reinforcement architecture can be designed to change the shape of composites upon diverse external stimuli, we first present shape-changing mechanisms in selected natural systems. A synthetic procedure that enables replication of these principles in artificial composites is then described and eventually used to produce artificial composites that bend and/or twist when hydrated. Finally, the uniqueness of the proposed approach is demonstrated by creating bulk samples that can undergo multiple, reversible shape changes upon the application of both humidity and temperature, and by producing monolithic composites in which multiple types of shape change are locally programmed within the same material. Reinforcement architecture in seed dispersal units that bend The pinecone closes its scales upon hydration and then reopens them upon dehydration [16] , [17] ( Fig. 1a , Supplementary Movie 1 ). This shape change can be linked to the local CMF orientation within the scale. The pinecone scale is a bilayer comprised roughly of a lower section with strong reinforcement perpendicular to the long axis of the scale and an upper section exhibiting reinforcement along the long axis of the scale [17] . This is presented in a very simplified cartoon in Fig. 1c just to convey the basic reinforcement architecture to the reader [20] . In reality, CMF alignment has a degree of randomization and the multilamellar wall of plant cells are far more complex than depicted in this simplified cartoon. Owing to the orientation of the CMFs in the two sections, the top section is reinforced against swelling along the scale’s long axis while the bottom section is not. As the two layers are tightly connected, barring any possibility of delamination, the hydrating scale exists in a frustrated configuration with the bottom section attempting to expand yet fixed to the reinforced top section. The minimal energy configuration is for the scale to bend, allowing maximum expansion for the bottom region along the long axis while minimizing swelling in the top region. A similar CMF architecture and bending mechanism is found in the wheat awn structure, which spreads open when dehydrated and closes again upon hydration [9] ( Fig. 1f ). Each side of the wheat awn is comprised of an inner cap with CMFs aligned along the long axis of the awn and an outer ridge with random CMF orientation ( Fig. 1h ). This randomness gives the ridge a slightly higher degree of swellability along the long axis of the awn as compared with the cap causing the wheat awn to close upon swelling. Reinforcement architecture in seed dispersal units that twist The seedpod of orchid trees, such as Bauhinia variegata , opens with its two halves twisting helically away from each other when drying [18] ( Fig. 1k ). The helical twisting is again the result of the CMF architecture. Each half of this chiral seedpod is comprised of a bilayer structure with outer and inner layers reinforced by CMF. If the long axis of the seedpod is at an angle of π /4 (to be consistent with subsequent designations), then the CMFs in each layer are predominantly angled at 0 and π /2 ( Fig. 1m ). This perpendicular configuration is enough to drive flat to helically shape change upon hydration. Both seedpod layers desire to expand perpendicular to the other causing a frustrated geometry. The shape providing the minimum frustration energy is a helical twist as observed in a drying seedpod [18] . Interestingly, such bilayer architecture allows for both twisting and bending depending upon the relationship between the CMF orientation and the long axis of the seedpod. For example, if a strip of the seedpod is extracted at an angle of π /2, the seedpod will behave as the pinecone scale and bend. At an intermediate angle, the seedpod will combine twisting and bending. Production of bulk hygroscopic composites with deliberate reinforcement architectures To simulate the shape-changing reinforcing effect of CMFs, we employ 7.5 μm diameter, 200-nm-thick aluminium oxide platelets with an estimated tensile strength of a few GPa. Such platelets have a distinct geometry relative to CMFs, offering 2D reinforcement compared with the 1D reinforcement of fibres. Thus, low or high CMF angle reinforcement can be recreated simply with horizontally or vertically oriented platelets, respectively, with respect to the long axis of the object ( Supplementary Figure S1 ). To gain control over the orientation of these microplatelets, 12-nm-diameter superparamagnetic iron oxide nanoparticles were adsorbed onto the platelet surface electrostatically [21] . As the nanoparticles are on the outside of the platelet in position to maximize torque, these coated platelets exhibit a UHMR effect enabling facile orientation under low external magnetic fields. Uniform magnetic fields thus pin one of the long axes of the platelets axially parallel to the field direction. In addition, the second long axis can be fixed by employing rotating magnetic fields of sufficiently high rotational frequency [21] , [22] . Bulk hygroscopic composites were produced by mixing UHMR alumina platelets into fluid polymer solutions that were then allowed to gel in the presence of a magnetic field. Various polymers were investigated, including gelatin, poly( N -isopropylacrylamide) (PNIPAAM) and alginate. Both monolayer and bilayer composites exhibiting deliberate alignment of reinforcement particles were produced by depositing one and two consecutive layers, respectively. The basic concept of constrained swelling/shrinking in the direction of the reinforcement was investigated for monolayers with horizontally and vertically aligned reinforcement arrangements in gelatin and alginate systems. Monolayers containing 7.5 vol% aligned alumina platelets show 250% higher swelling and 200% higher shrinkage in the direction perpendicular versus parallel to the reinforcement axes for swelled gelatin and for cross-linked alginate, respectively ( Supplementary Figures S2,S3 and Supplementary Movie 2 ). Such constrained swelling in the reinforcement direction was exploited to form bioinspired bilayers that bend and/or twist depending on the programmed reinforcement architecture, as described below. Synthetic hygroscopic composites that bend The bilayer configurations exhibited by the pinecone ( Fig. 1a–c ) and by the wheat awn structure ( Fig. 1f–h ) were replicated artificially to obtain gelatin–alumina composites that bend upon drying/hydration. To mimic the pinecone architecture, 7.5 vol% UHMR alumina platelets were aligned with the help of a rotating magnet following the two-step process schematically illustrated in Fig. 2 . A similar procedure was used to obtain bilayers that replicate the wheat awn structure, except that in this case no magnetic field was applied during preparation of the first layer in order to reproduce the random outside reinforcement architecture consistent with this natural system (II in Fig. 1h ). Drying of synthetic hydrogels mimicking the pinecone scales caused bending of the composite towards the layer exhibiting reinforcement orientation perpendicular to the bilayer’s long axis ( Fig. 1d ). Hydration makes this same layer strongly expand and thus bend the scale into the opposite curvature ( Fig. 1e , Supplementary Movie 3 ). Such a response follows precisely the autonomous hygroscopic actuation of the natural pinecone and occurs at similar time scales. Similarly, the slightly higher long-axis swellability of the outside layers of the synthetic wheat awn structure makes them close upon hydration. If dried, the wheat awn system spreads open again ( Fig. 1i , Supplementary Movie 4 ). This reversible bending response is similar in nature to that of bimetallic thermostats and of a family of synthetic bilayer structures comprised of two distinct materials [7] , [20] , [21] . 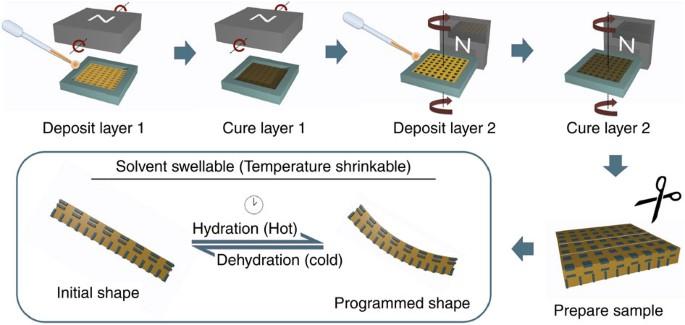Figure 2: Typical manufacturing method used to create bioinspired self-shaping reinforced composites. A hydrogel solution containing Al2O3platelets coated in iron oxide nanoparticles is added to a Teflon mould above which a rare-earth permanent magnet is rotated. The hydrogel is cured under the rotating field, preserving the orientation of the reinforcing platelets. To form a bilayer structure, a second hydrogel solution containing platelets is added to the mould and a different magnetic field is applied. To mimic a horizontal rotating field, the mould can instead be rotated adjacent to a static permanent magnet as depicted. The second layer of the hydrogel is then cured preserving a different orientation of reinforcing platelets. The bilayer can then be removed from the mould and prepared as desired. As depicted in the box, swelling/shrinkage of the polymer matrix upon external stimuli make these hydrogels reversibly change shape guided by the orientation of the reinforcement platelets. For certain materials (for example, gelatin), the reinforced hydrogels can be swelled in the presence of a solvent (for example, water) to drive a shape change. In other materials (for example, PNIPAAM), the reinforced hydrogels can be shrunk upon increase of the system’s temperature (for example, T>35 °C). In both cases, these shape changes are reversible with the material returning to its initial shape upon either dehydration or cooling. Figure 2: Typical manufacturing method used to create bioinspired self-shaping reinforced composites. A hydrogel solution containing Al 2 O 3 platelets coated in iron oxide nanoparticles is added to a Teflon mould above which a rare-earth permanent magnet is rotated. The hydrogel is cured under the rotating field, preserving the orientation of the reinforcing platelets. To form a bilayer structure, a second hydrogel solution containing platelets is added to the mould and a different magnetic field is applied. To mimic a horizontal rotating field, the mould can instead be rotated adjacent to a static permanent magnet as depicted. The second layer of the hydrogel is then cured preserving a different orientation of reinforcing platelets. The bilayer can then be removed from the mould and prepared as desired. As depicted in the box, swelling/shrinkage of the polymer matrix upon external stimuli make these hydrogels reversibly change shape guided by the orientation of the reinforcement platelets. For certain materials (for example, gelatin), the reinforced hydrogels can be swelled in the presence of a solvent (for example, water) to drive a shape change. In other materials (for example, PNIPAAM), the reinforced hydrogels can be shrunk upon increase of the system’s temperature (for example, T>35 °C). In both cases, these shape changes are reversible with the material returning to its initial shape upon either dehydration or cooling. Full size image Synthetic hygroscopic composites that twist In addition to simple bending, the composite reinforcement architecture can also be designed to cause a hydration-driven twisting action that is not possible in simple synthetic bilayer materials. As illustrated in the orchid tree seedpod, twisting can be achieved if the reinforcing elements are not only orthogonally arranged within the bilayer (as in bending seed dispersal units) but are also oriented with an angle of π /4 with respect to the pod’s long axis ( Fig. 1k–m ). Synthetic composites with such bioinspired twisting architecture were produced and subjected to drying/hydration cycles. The results show that as the two layers attempt to expand in perpendicular directions during hydration, the frustrated system is driven to chirally twist similar to the natural response ( Fig. 1n , Supplementary Movie 5 ). Drying of the twisted hydrogel brings the structure back to its original flat geometry ( Supplementary Movie 6 ). Both left-handed and right-handed twisting can be achieved by simply changing the sequence of the angles of the applied magnetic field from 0: π /2 to π /2: 0. To demonstrate that the rich combination of twisting and bending motions achievable in materials extracted from orchid tree seedpods [18] can also be implemented in synthetic composites, we cut samples from an artificial orchid tree seedpod bilayer at varying angles between − π /2 and +π/2 ( Fig. 3 ). A clear transition from bending to twisting is indeed observed upon hydration of the synthetic bilayers ( Fig. 3a–c , Supplementary Figure S4 and Supplementary Movies 5–7 ). 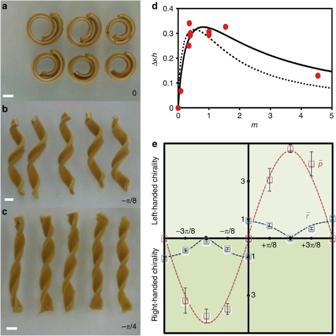Figure 3: Shape change in synthetic monolithic materials that mimic reinforcement orientations of a chiral seedpod. (a–c) Synthetic materials with bilayer reinforcement architectures orientated at 0 andπ/2 mimicking the orientation of an orchid tree seedpod (Fig. 1m) and removed at a cutting angle of (a) 0, (b) –π/8 or (c) –π/4. (d) With a cutting angle of 0 orπ/2, the material undergoes pure bending with a final predictable curvature that depends very strongly on the thickness ratio of the two reinforcement layers (m). Experimental data (dots) are well described by theoretical predictions (lines) from Equation 1. Dotted line is consistent with strain measurements of gelatin monolayers (n=3.53), while solid line is best fit (n=1.50). (e) With equal thickness of the two layers, normalized material curvature,, and normalized pitch,, show a strong dependence upon the cutting angle. Results are in good agreement with the theoretical predictions (dashed lines) for the orchid tree seedpod18. Figure 3: Shape change in synthetic monolithic materials that mimic reinforcement orientations of a chiral seedpod. ( a – c ) Synthetic materials with bilayer reinforcement architectures orientated at 0 and π /2 mimicking the orientation of an orchid tree seedpod ( Fig. 1m ) and removed at a cutting angle of ( a ) 0, ( b ) – π /8 or ( c ) – π /4. ( d ) With a cutting angle of 0 or π /2, the material undergoes pure bending with a final predictable curvature that depends very strongly on the thickness ratio of the two reinforcement layers ( m ). Experimental data (dots) are well described by theoretical predictions (lines) from Equation 1. Dotted line is consistent with strain measurements of gelatin monolayers ( n =3.53), while solid line is best fit ( n =1.50). ( e ) With equal thickness of the two layers, normalized material curvature, , and normalized pitch, , show a strong dependence upon the cutting angle. Results are in good agreement with the theoretical predictions (dashed lines) for the orchid tree seedpod [18] . Full size image Quantitative prediction of shape change of synthetic hygroscopic composites Quantitative predictions of the effects of the initial reinforcement architecture on the final geometry of the object after swelling/shrinkage are essential to create a ‘programming code’ for deliberate control of the composite shape change. To establish predictive structure–function relationships for bending bilayer composites that mimic pinecone and orchid tree seedpod architectures with cutting angles at 0 or π /2, we investigated the influence of the relative thickness, m , between individual layers on the final curvature, κ 0 , of a bent object after swelling in water ( Fig. 3a ). The object curvature was found to be strongly affected by the thickness ratio m , with a maximum observed when the passive layer is approximately half the thickness of the active layer ( Fig. 3d ). These results can be explained with the help of the theory for bimetallic thermostats [16] , [23] , which predicts the following dependence of the thickness-normalized bilayer curvature, Δκh , on the thickness ratio m : where n is the ratio between the elastic moduli of the passive and active layer in the long-axis direction ( E p / E a ), m is the ratio between the thickness of the passive horizontally reinforced layer and the thickness of the active vertically reinforced layer, h p / h a , and h is the total thickness of the bilayer. Our experimental data were observed to follow the same trend predicted by the theory for bimetallic thermostats [16] , [23] , if we assume n to vary between 1.50 (best fit, solid line) and 3.53 (obtained from independent monolayer experiments, dotted line, Supplementary Figure S2 ) ( Fig. 3d ). In addition to the good agreement between experimental points and Equation (1), the range of n values obtained compares well with the increase in elastic modulus of the polymer matrix upon platelet addition seen in previous studies. The reinforcement factor n typically lies within the range 1.3–3.0 for composites containing the volume fraction of platelets of 7.5 vol% used in these experiments [24] , [25] . To investigate the programmability of the transition between twisting and bending within synthetic composites that mimic orchid tree seedpod architectures, various cutting angles were investigated from − π /2 to + π /2. Both the normalized radius of curvature, = rκ 0 , and the normalized pitch length, = pκ 0 , were monitored during swelling of the synthetic composites. Here, r is the radius of the encompassing cylinder of the twisting composite strip and p is the pitch length. κ 0 , the reference curvature, was determined by measuring the average swollen curvature of very thin strips of composites at cutting angles of 0 and π /2. The normalized radius of curvature and pitch are found to follow the same trends expected from theoretical predictions proposed to describe the hydration responses of the natural orchid tree seedpod ( Fig. 3e ) [18] . This indicates that a balance between the bending and stretching energies that develop during the swelling process determines the mechanical behaviour of the synthetic composites. The experimentally obtained data match exactly the predicted values, while the normalized pitch is quantitatively well described by the theory if adjusted by a scaling factor of 0.7. This scaling factor indicates that the synthetic composites created exhibit a stronger response in twisting compared with bending that can possibly be attributed to gravitational effects. Still, our ability to quantitatively predict the final shape of the composites based on their initial geometrical features makes this a powerful approach to achieve tailored, programmable shape changes using synthetic materials. Multiresponsive self-shaping composites As the proposed method relies primarily on the microstructure of the composite rather than on the specific chemistry of its constituent building blocks, any kind of swellable/shrinkable matrix that responds to external stimuli can be used to trigger the shape change. To illustrate the generality of this approach and the possibility to extend it to other stimuli-responsive matrices, PNIPAAM–alumina hydrogels that mimic the orchid tree seedpod structure were investigated as an example of a bilayer composite that self-shapes not only in response to hydration but also to temperature changes. Owing to the temperature-triggered shrinkage of the PNIPAAM hydrogel and the programmed orientation of the reinforcement particles within the matrix, the composite was driven to helically twist upon increasing the water’s temperature above 35 °C ( Fig. 4b ). By decreasing the water temperature to 25 °C, the hydrogel expanded and returned to its straightened state ( Fig. 4c ). To probe the secondary hydration-driven mechanism, the PNIPAAM–alumina composite was allowed to swell in the water bath overnight. This swelling drove the composite to helically twist in the opposite direction. Therefore, by oscillating both temperature and hydration levels the sample could be changed from exhibiting left-handed chirality to showing right-handed chirality. Such oscillation was found to be robust and reversible over more than 20 cycles ( Supplementary Figure S5 ). 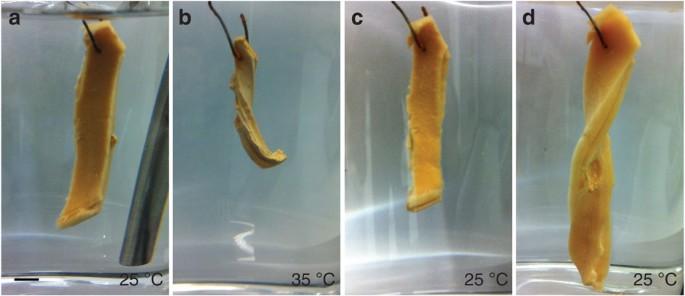Figure 4: Reinforced PNIPAAM dual stimuli system that twists in different directions depending on the external trigger. (a) A PNIPAAM hydrogel containing two layers of 5 vol% Al2O3platelets oriented in the chiral seedpod configuration (Fig. 1m). Water temperature is first kept at 25 °C. (b) The PNIPAAM hydrogel undergoes a large shrinkage upon increasing the system temperature beyond 35 °C, which causes the rectangular bilayer to chirally twist. (c) Upon cooling the system back to 25 °C, the material returns to its original shape. (d) Maintaining room temperature, the PNIPAAM hydrogel swells beyond the as-prepared geometry causing a chiral twist in the opposite direction. Scale bar is 500 μm. Figure 4: Reinforced PNIPAAM dual stimuli system that twists in different directions depending on the external trigger. ( a ) A PNIPAAM hydrogel containing two layers of 5 vol% Al 2 O 3 platelets oriented in the chiral seedpod configuration ( Fig. 1m ). Water temperature is first kept at 25 °C. ( b ) The PNIPAAM hydrogel undergoes a large shrinkage upon increasing the system temperature beyond 35 °C, which causes the rectangular bilayer to chirally twist. ( c ) Upon cooling the system back to 25 °C, the material returns to its original shape. ( d ) Maintaining room temperature, the PNIPAAM hydrogel swells beyond the as-prepared geometry causing a chiral twist in the opposite direction. Scale bar is 500 μm. Full size image Monolithic composites with programmable site-specific shape changes Because of its microstructural origin, the shape change mechanism investigated here also offers the possibility to program multiple bending and/or twisting movements at different sites of the same monolithic composite. This can be accomplished by locally tuning the orientation of UHMR platelets within specific regions of the continuous polymer matrix. The modular nature of this approach and the full orientational control offered by the UHMR platelets open the possibility to design and create completely unique and programmable shape changes that are not observed in nature. As illustrative examples, monolayer and bilayer gelatin–alumina composites were produced exhibiting distinct modular regions of platelets aligned at specific angles with respect to the specimen’s long axis ( Fig. 5a ). Hydration of these systems leads to different local deformations of the sections, with a 50% larger strain in the direction perpendicular to the reinforcement long axis ( Fig. 5b ). To obtain self-shaping materials exhibiting distinct twisting and bending sections, a gelatin–alumina bilayer composite was created that had three regions: (I) chiral twisting, (II) leftward bending and (III) rightward bending, ( Fig. 5d–f , Supplementary Movie 8 ). By combining regions of twist with regions of bend, a limitless number of programmable shape change configurations are enabled. 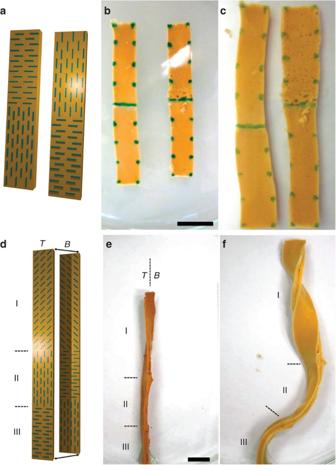Figure 5: Programming of the local reinforcement orientation to achieve site-specific shape changes in synthetic materials. (a) A cartoon schematic of a possible monolayer reinforcement architecture produced in (b) an alumina–gelatin composite. (c) Swelling of such a system leads to shape change in correspondence with the local reinforcement architecture. The gelatin matrix swells 50% more in the direction perpendicular to the local reinforcement orientation. (d) A cartoon schematic of a possible bilayer structure produced in (e) an alumina–gelatin bilayer composite. (f) Swelling of the bilayer system leads to local regions that curl or twist depending upon the previously programmed reinforcement architecture. Scale bar, 1 cm. Figure 5: Programming of the local reinforcement orientation to achieve site-specific shape changes in synthetic materials. ( a ) A cartoon schematic of a possible monolayer reinforcement architecture produced in ( b ) an alumina–gelatin composite. ( c ) Swelling of such a system leads to shape change in correspondence with the local reinforcement architecture. The gelatin matrix swells 50% more in the direction perpendicular to the local reinforcement orientation. ( d ) A cartoon schematic of a possible bilayer structure produced in ( e ) an alumina–gelatin bilayer composite. ( f ) Swelling of the bilayer system leads to local regions that curl or twist depending upon the previously programmed reinforcement architecture. Scale bar, 1 cm. Full size image In summary, synthetic hydrogel composites that can self-shape into programmed configurations upon external stimuli were created using the bending and twisting mechanisms exhibited by pinecones, wheat awn structures and orchid tree seedpods. In contrast to state-of-the-art shape-memory alloys and synthetic multilayered films, the proposed self-shaping composites generate shape change through the purposeful local orientation of reinforcing platelets throughout monolithic structures. Such bioinspired architecture can be recreated in synthetic systems by controlling the orientation of UHMR microplatelets using low magnetic fields. Relying on microstructural design rather than on the specific chemistry of the constituent materials, the shape-changing mechanism outlined here is potentially applicable to any composite system comprising of anisotropic reinforcing elements surrounded by a matrix that undergoes significant dimensional changes upon a given external stimuli, opening several new possibilities for the design of composite materials with unusual self-shaping features. Preparation of UHMR platelets To obtain UHMR anisotropic particles, 37.5 μl of anionic ferrofluid (EMG-705, Ferrotec, Germany) per gram of alumina platelets desired were diluted into 40 ml of deionized water and were immediately added dropwise to a suspension of alumina platelets (AlPearl −7.5 μm, Antaria, Bentley, Australia) in 300 ml of deionized water under vigorous stirring. The pH was held at 7 to keep a net positive charge on the surface of the alumina platelets. The anionic surfactant of the EMG-705 ferrofluid enables thus the electrostatic adsorption of the iron oxide superparamagnetic nanoparticles onto the surface of the alumina platelets. Adsorption was determined to be complete when the supernatant was optically clear. The platelets were then filtered and dried at 150 °C for 16 h. Synthesis of the gelatin–alumina hydrogels Gelatin–alumina hydrogel composites were produced by mixing UHMR alumina platelets into a molten 20 vol% gelatin aqueous solution at 45 °C (gelatin from porcine skin, Sigma-Aldrich). The solution was poured into a glass mould and subjected to a rotating magnetic field. To simulate out-of-plane reinforcement, a 5 cm × 5 cm × 2 cm rare-earth magnet (Supermagnete, Switzerland) was rotated with a rotary drill above the mould in the first arrangement shown in Fig. 2 . For in-plane reinforcement, the permanent magnet was held in place, while the glass mould was rotated as depicted in the second arrangement shown in Fig. 2 . As the gelatin cooled, the tropocollagen molecules form triple helices via hydrogen bonds that serve to cross-link the hydrogel. After cooling for 10 min to 25 °C, the gelatin–alumina hydrogel composite can be removed from the mould, cut to length and experimentally tested. For the synthetic pinecone configuration, a first layer of gelatin–alumina was deposited under a vertically rotating magnetic field followed by a second layer under a horizontally rotating magnetic field ( Fig. 2 ). The second molten layer melts the surface of the first layer to provide a good interfacial connection between them, preventing delamination. The sample was then cut into eight 1–2 cm strips and each were glued to a glass support rod ( Fig. 1d ). Synthetic wheat awn structures were produced by first depositing a layer of gelatin–alumina without an external magnetic field. This led to the random reinforcement orientation of the wheat awn ridge (region II in Fig. 1h ). A second layer was then deposited under a horizontally rotating magnetic field to produce the awn’s cap (region I in Fig. 1h ). Two 1 × 4 cm 2 sections were cut from the hydrogel and glued to a glass substrate ( Fig. 1i ). To produce synthetic composites with the orchid tree seedpod architecture, a first gelatin–alumina layer was deposited under a vertically rotating magnetic field at an angle of 0 to the main axis of a glass mould. A second layer was added after switching the magnetic field to rotate at an angle of π /2. The resulting sample was cut into a 1 × 6 cm strip with the long axis along + π /4 and submerged in water to swell upon hydration. For swelling experiments, the hydrogel composites were placed on a small metal hanger to fully submerge them in deionized water and observed over time. Synthesis of the PNIPAAM–alumina hydrogels Each layer of the PNIPAAM–alumina composites was created by mixing NIPAAM with a thickening agent, cross-linker, initiator, accelerator and 10 vol% UHMR platelets. The layers were made sequentially being polymerized under distinct applied magnetic fields. The second layer was polymerized while in contact with the first, leading to strong lamination likely as a result of interdiffusion of a small fraction of monomer and cross-linker species. For each layer of the PNIPAAM–alumina bilayer hydrogel, 500 μl of a 25 wt% NIPAAM (monomer) aqueous solution was mixed with 500 μl of a 2 wt% methyl cellulose (thickening agent) aqueous solution and 50 μl of 0.5 wt% N , N ′-methylenebisacrylamide (cross-linker) aqueous solution. Four hundred milligrams of UHMR platelets were mixed thoroughly into the solution. Then, 70 μl of a 1 wt% ammonium persulfate (initiator) aqueous solution, 200 μl of a 2 wt% tetramethylethylenediamine (accelerator) aqueous solution and 170 μl of deionized water were added. The resulting suspension was homogenized and pipetted into a 2.3 cm × 2.1 cm × 1 mm PTFE mould until the mould was filled. For the first layer, the mould was covered with a glass slide to produce a flat, uniform film and placed in vertical rotating magnetic field at an angle of 0, as shown in Fig. 1 . Polymerization took place in about 10 min. For the second layer, the mould was filled with fresh suspension and covered with the first PNIPAAM–alumina hydrogel layer that was stuck to a glass slide. A spacer was used to adjust the relative height between the first and second gels. The mould was placed in a vertical rotating magnetic field at an angle of + π /2. Polymerization again took ~10 min. The hydrogel was removed and rinsed extensively in deionized water. A 0.5 × 2.5 cm 2 section was removed with a cutting angle of + π /4 and soaked in deionized water for observation ( Fig. 4a ). Synthesis of the alginate–alumina hydrogels Alginate–alumina hydrogels were produced by mixing 5 vol% UHMR alumina platelets into a 4 wt % aqueous alginate solution (Alginic Acid, Sigma-Aldrich). Four hundred microlitres of alginate solution was poured into a circular plastic mould with a diameter of 12 mm. A horizontal or vertical rotating magnetic field was applied to produce in-plane and out-of-plane reinforcement, respectively. The fluid alginate composites were then carefully submerged quickly into 1 ml of 20 wt% CaCl 2 solution that lead to rapid cross-linking of the alginate molecules with Ca +2 ions. Such cross-linking leads to dramatic volume reduction of the composite that can be guided by the orientation of the reinforcement particles ( Supplementary Figure S3 ). Analysis of the twisting and bending movements To quantify the level of twisting and bending in the self-shaping composites, photographs of the programmed structures were taken over time. These photographs were then analysed in ImageJ (NIH, USA) to measure lengths, determine bending curvatures and calculate twisting angles. Synthesis of monolithic composites with programmable site-specific shape changes These materials were made using the above synthesis protocol for gelatin–alumina composites in a stepwise process, allowing curing of the gel in each region under the appropriate magnetic field. In the monolayer example, 0.5 × 4 cm 2 films were produced with one half containing reinforcement aligned parallel to the long axis and the other half with reinforcement oriented perpendicular to the long axis ( Fig. 5a ). In the twisting/bending bilayer example, a 0.7 × 7 cm 2 film was produced in six consecutive steps programming the architecture of each layer in regions I, II and III in the configurations indicated in Fig. 5d . Analogy between reinforcement architectures in synthetic and natural composites Alumina platelets at deliberate orientations were used in this study to mimic the reinforcement architecture of CMFs within the wall of plant cells. Supplementary Figure S1 illustrates the analogy between these two systems. How to cite this article: Erb, R.M. et al . Self-shaping composites with programmable bioinspired microstructures. Nat. Commun. 4:1712 doi: 10.1038/ncomms2666 (2013).